Genome dynamics of the human embryonic kidney 293 lineage in response to cell biology manipulations The HEK293 human cell lineage is widely used in cell biology and biotechnology. Here we use whole-genome resequencing of six 293 cell lines to study the dynamics of this aneuploid genome in response to the manipulations used to generate common 293 cell derivatives, such as transformation and stable clone generation (293T); suspension growth adaptation (293S); and cytotoxic lectin selection (293SG). Remarkably, we observe that copy number alteration detection could identify the genomic region that enabled cell survival under selective conditions (i.c. ricin selection). Furthermore, we present methods to detect human/vector genome breakpoints and a user-friendly visualization tool for the 293 genome data. We also establish that the genome structure composition is in steady state for most of these cell lines when standard cell culturing conditions are used. This resource enables novel and more informed studies with 293 cells, and we will distribute the sequenced cell lines to this effect. The human embryonic kidney (HEK) 293 cell line and its derivatives are used in experiments ranging from signal transduction and protein interaction studies over viral packaging to rapid small-scale protein expression and biopharmaceutical production. The original 293 cells [1] , [2] , [3] were derived in 1973 from the kidney of an aborted human embryo of unknown parenthood by transformation with sheared Adenovirus 5 DNA. The human embryonic kidney cells at first seemed recalcitrant to transformation. After many attempts, cell growth took off only several months after the isolation of a single transformed clone. This cell line is known as HEK293 or 293 cells (ATCC accession number CRL-1573). A 4-kbp adenoviral genome fragment is known to have integrated in chromosome 19 (ref. 4 ) and encodes for the E1A/E1B proteins, which interfere with the cell cycle control pathways and counteract apoptosis [5] , [6] . Cytogenetic analysis established that the 293 line is pseudotriploid [7] . Given the broad use of 293 cells for biomedical research and virus/protein production, we decided to perform a comprehensive genomic characterization of the 293 cell line and the most commonly used derived lines ( Fig. 1a ) to better understand the dynamics of the 293 genome under the procedures commonly used in biotechnological engineering of mammalian cell lines. 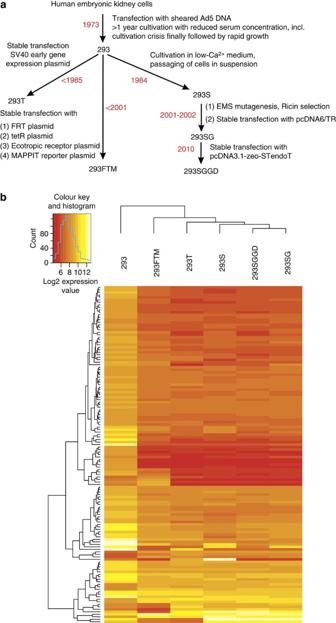Figure 1: HEK293 cell line expression profiling. (a) Schematic overview of the studied 293 cell lines and their derivation history. FRT plasmid: pFRT/lacZeo; TetR plasmid: pcDNA6/TR; ecotropic receptor plasmid: pM5neo-mEcoR; MAPPIT reporter plasmid: pXP2d2-rPAP1-luci. (b) Heatmap of the 136 genes differentially expressed in every cell line when compared with the 293 line. Colour-coded values represent the log2expression values after summarization, normalization and averaging over three biological replicates per cell line. Genes (rows) and cell lines (columns) were clustered hierarchically according to similarity between expression levels. See alsoSupplementary Figs 6–8. Figure 1: HEK293 cell line expression profiling. ( a ) Schematic overview of the studied 293 cell lines and their derivation history. FRT plasmid: pFRT/lacZeo; TetR plasmid: pcDNA6/TR; ecotropic receptor plasmid: pM5neo-mEcoR; MAPPIT reporter plasmid: pXP2d2-rPAP1-luci. ( b ) Heatmap of the 136 genes differentially expressed in every cell line when compared with the 293 line. Colour-coded values represent the log 2 expression values after summarization, normalization and averaging over three biological replicates per cell line. Genes (rows) and cell lines (columns) were clustered hierarchically according to similarity between expression levels. See also Supplementary Figs 6–8 . Full size image First among these derived lines, we analysed 293T, which expresses a temperature-sensitive allele of the SV40 T antigen [8] , [9] . This enables the amplification of vectors containing the SV40 ori and thus considerably increases the expression levels obtained with transient transfection. SV40 T forms a complex with and inhibits p53, possibly further compromising genome integrity [10] . The original 293 line was suspension growth-adapted through serial passaging in Joklik’s modified minimal Eagle’s medium [11] . Full adaptation took about 7 months, and the first passages were so difficult that the few cells that grew through are likely to have been almost clonal (Dr Bruce Stillman, personal communication). The fully adapted cell line is known as 293S and is also analysed here. Subsequently, this line was mutagenized with ethylmethanesulfonate (EMS) and a Ricin toxin-resistant clone was selected out. The line lacked N-acetylglucosaminyltransferase I activity (encoded by the MGAT1 gene) and accordingly predominantly modifies glycoproteins with the Man 5 GlcNAc 2 N-glycan. Then, a stable tetR repressor–expressing clone of this glyco-engineered cell line was derived to enable tetracyclin-inducible protein expression [12] . This cell line is widely used for the production of homogenously N-glycosylated proteins and will be referred to as 293SG. Apart from these four cell lines in common use, we also analysed the genome of two 293-derived lines used in our laboratory for protein–protein interaction screening (293FTM) and glyco-engineering (293SGGD; details in Supplementary Information ). In our study, following genomic studies of other human cell lines [13] , [14] , [15] , we aim to provide a full-genome resource for these cell biology ‘workhorse’ cell lines while developing the necessary tools to make such resources easily available. This enables all researchers using the 293 cell lines to make fully informed analyses of genomic regions of interest to their studies, without expert bioinformatics skills. We also map the genomic changes accumulating after standard laboratory cell culturing (passaging and freezing), providing a way to assess genomic stability of each line. Furthermore, we present a workflow for determining the insertion sites of viral sequences and plasmids based on the genome sequencing data. The extreme chromosome structure diversity/plasticity in the 293 cell line underlies a novel application: selection of 293 clones surviving stringent selective conditions (in our case: ricin toxin), followed by whole-genome analysis of copy number alterations, can effectively pinpoint the genomic region(s) that contain the gene(s) that is required for adaptation to those selective conditions. 293 cell lineage genome, karyotype and transcriptome For genome resequencing, we used complete genomics (CG) high-coverage genome sequencing technology [16] ( Supplementary Methods ; data set summary in Supplementary Tables 1 and 2 , and sequencing quality overview in Supplementary Fig. 1 ). 293 cells are of female provenance, as we find no trace of Y-chromosome-derived sequence in our data sets. The mitochondrial sequence belongs to the oldest European haplogroup U5a1 (refs 17 , 18 ). Furthermore, we applied multiplex fluorescence in situ hybridization analysis to our 293 lines ( Supplementary Data 1 ). A wide diversity of karyotypes was found, also within each clone, with some chromosomal alterations relative to the human reference genome present in almost all cells, and others in only a small proportion of cells. Overall, the pseudotriploidy of the 293 lineage was confirmed both by CG sequencing and karyotyping. To further define the 293 cell lineage and to enable the future development of cell line authentication genotyping assays, we analysed which single-nucleotide polymorphisms (SNPs) in protein-coding regions were common to the six sequenced 293 cell lines ( Supplementary Data 2 ) and we manually curated the functional annotation of all novel (that is, not present in dbSNP) 293-defining SNPs ( Supplementary Data 2 ). The genome-wide 2-kb-resolution sequencing coverage depth analysis provides a 2-kb-window copy number that is relative to the genome-averaged copy number in that particular genome. To obtain the absolute copy number, an independent data source is required. For this purpose, we used the Illumina SNP-array-determined genome-averaged ploidy number. The resulting calibrated 2-kb-resolution copy number shows very good consistency with the lower-resolution Illumina SNP-array copy number variant (CNV) results (Spearman rho=0.67–0.80, depending on the cell line; P <2.2e−16) and reveals that the 293 cell genome is characterized by a large number of CNVs, which, together with the heterogenous karyotyping results, paints the picture of a genome that is evolving through a process of frequent chromosomal translocations involving most of the genome. The absolute 2-kb-resolution copy number was integrated in our 293 genome browsers (see below). An overview of genome-wide CNVs for a normal human genome and for each of the 293-derived cell lines is provided in Supplementary Fig. 2 , and more detail per chromosome is provided in Supplementary Data 3 . From the CG sequencing data, we also derived the B-allele frequency (BAF) for all of the SNPs and averaged those over 10-kbp bins ( Supplementary Fig. 3 ). These data allow for interpretation of the ploidy level in terms of the number of copies of the different alleles that are present (including loss of heterozygosity) and further lend some support to the ploidy level call (for example, a BAF of 0.33 in a triploid region indicates one copy of one parental allele and two copies of the other). However, it should be noticed that both copy number and BAF obtained here are weighted averages of these values over the distribution of karyotypes within each cell line. For example, in some cases a presence of an allele at 0.6 copies per genome is calculated (0.2 BAF in a triploid region). In light of the karyotypic diversity within the cell lines, that should be interpreted as heterogeneity in the cells, some of which will have loss of heterozygosity for that region (0 copies of that allele) and some of which will have retained one copy. Subsequently, to establish the phenotypic characteristics of the different sequenced 293-derived cell lines, we profiled the transcriptome of each cell line with exon arrays. Genome and transcriptome data were integrated with the data derived thereof in the IGV browser interface (see below). There is some controversy as to the likely embryonal cell type from which 293 cells have arisen: the line was derived from embryonic kidney and some evidence exists to suggest a neuronal lineage [19] . We have extracted cell-type-specific gene expression signatures from Genevestigator [20] for adrenal tissue, kidney, central nervous tissue and pituitary tissue, and intersected these with the transcriptome of 293 cells, followed by Ingenuity Pathway Analysis (IPA) of the intersection ( Supplementary Fig. 4 and Supplementary Table 3 ). 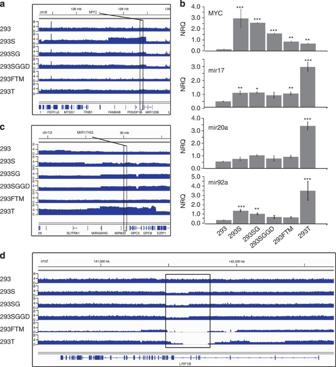Figure 3: Notable amplifications and deletions in 293 cell lines. (a) On the q-arm of chromosome 8, the 293S line shows an amplification of a 1.6-Mb region containing theMYClocus. The 293SG and 293SGGD lines seem to have partially lost this rearrangement. (b) Expression validation by quantitative real-time PCR forMYCand three microRNAs from the polycistronicMIR17HGlocus (mir17, mir20a and mir92a, respectively). Expression levels of these microRNAs are markedly higher in 293T than in any of the other 293 lines (fold change between 2.5 and 8.8). Values are represented as normalized relative quantities (NRQ)±s.e.m. (n=3). Significantly different NRQs in comparison with the 293 line are indicated as *Pvalue<0.05, **Pvalue<0.01, ***Pvalue<0.001 and were analysed using a one-way analysis of variance with a Tukey HSDpost hoctest. (c) Similarly, theMIR17HGgene is located in an extended amplified region on chr13 in the 293T cell line, where copy numbers reach up to 8. (d) Part of the LRP1B gene—comprising exons 3–7 (300 kb) or 4–7 (400 kb)—has been deleted in the 293FTM and 293T line. Copy numbers downstream of this region are also reduced in 293FTM. See alsoSupplementary Fig. 5for another notable deletion (including fumarate hydratase, found in all investigated 293 cell lines). In panelsa,candd, the Y-axis represents the genomic copy number. Whereas it is clear that 293 cells are transformed cells that have only limited transcriptional profile overlap with any of these mature tissue signatures, it is also evident that an adrenal lineage is the most likely among the three. The same conclusion was reached based on reanalysing the transcriptional profiling data in ref. 19 according to the same methodology. During embryonic development, the structure that will become the adrenal gland is prominently present adjacent to the kidney. The adrenal medulla is of neural crest ectodermal origin, which could explain the expression of some neuron-specific genes [19] . The hypothesis most in accordance with the available data would thus be an origin of the 293 cells in the embryonic adrenal precursor structure. Genomic and transcriptomic features of 293-derived cells 293 cell lines are known to have been transformed with an adenoviral sequence that integrated on chromosome 19 (ref. 4 and see below). A 332.5-kbp genomic region containing the adenoviral sequence insertion site has been amplified in all sequenced 293 cell lines: whereas the surrounding chr19 regions have a copy number of 3–4, this block of sequence has a copy number of 5–6 (depending on the 293 line, Fig. 2a ). 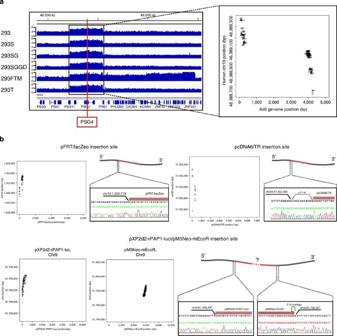In the face of the apparent constant genomic reshuffling in the 293 lineage, this finding suggests that positive selective pressure exists for the maintenance of a high copy number of the adenoviral sequence. Figure 2: Plasmid insertion site detection. (a) The Adenovirus 5 (Ad5) genome fragment is located in an 332.5-kb region on chr19 (48,221,000–48,553,500). This Ad5 sequence had been inserted and amplified in the 293 cell and the insertion and amplification have been maintained in thePSG4gene of the whole 293 lineage. The Y-axis represents the genomic copy number. The dot plot in the right panel shows individual paired-reads aligning on the Ad5 genome (xaxis) and chr19 (yaxis). (b) Detection and confirmation of plasmid insertion sites in the 293FTM cell line. Four plasmids have been inserted into this cell line. Note the 11 additional bases inserted upstream of the pcDNA/TR plasmid (right panel), as well as the likely tandem insertion of pXP2d2-rPAP1-luci and pM5Neo-mEcoR plasmids on chr9 (bottom panel). Notably, we were unable to validate the plasmid–plasmid breakpoint of pXP2d2-rPAP1-luci and pM5Neo-mEcoR, probably due to the presence of stretches of homologous sequence in both plasmid sequences. Black sequence: consensus of several trace files, green or red sequences: derived from the representative trace file below the sequence. See alsoSupplementary File 4. Figure 2: Plasmid insertion site detection. ( a ) The Adenovirus 5 (Ad5) genome fragment is located in an 332.5-kb region on chr19 (48,221,000–48,553,500). This Ad5 sequence had been inserted and amplified in the 293 cell and the insertion and amplification have been maintained in the PSG4 gene of the whole 293 lineage. The Y-axis represents the genomic copy number. The dot plot in the right panel shows individual paired-reads aligning on the Ad5 genome ( x axis) and chr19 ( y axis). ( b ) Detection and confirmation of plasmid insertion sites in the 293FTM cell line. Four plasmids have been inserted into this cell line. Note the 11 additional bases inserted upstream of the pcDNA/TR plasmid (right panel), as well as the likely tandem insertion of pXP2d2-rPAP1-luci and pM5Neo-mEcoR plasmids on chr9 (bottom panel). Notably, we were unable to validate the plasmid–plasmid breakpoint of pXP2d2-rPAP1-luci and pM5Neo-mEcoR, probably due to the presence of stretches of homologous sequence in both plasmid sequences. Black sequence: consensus of several trace files, green or red sequences: derived from the representative trace file below the sequence. See also Supplementary File 4 . Full size image Very strikingly, in all 293 lines, compared with the human RefSeq, the telomeric end of chromosome 1q is rearranged through deletions and inversions. This results in the loss of four out of five copies of the locus harbouring the fumarate hydratase gene ( Supplementary Fig. 5 ). This suggests that the 293 cells may be under selective pressure not to amplify the FH -containing region. Remarkably, most of the other citric acid cycle enzyme-coding genes conversely had a higher-than-average gene copy number in the 293 lineage ( Supplementary Data 4 ). Recent studies have implied the cytoplasmic fumarase in stabilization of the transcription factor HIF1α [21] , leading to a switch of the cellular energy metabolism from respiration to aerobic glycolysis accompanied with enhanced glutaminolysis [22] . Indeed, high glutamine consumption and ammonia and alanine production are well-known features of 293 cell fermentations [23] , [24] . Focal deletions in FH are associated with several types of cancer [25] ( http://www.broadinstitute.org/tumorscape/ ). Furthermore, we have carefully inspected all genes in the COSMIC (Catalogue Of Somatic Mutations In Cancer) database [26] , as well as genes involved in DNA repair and cell cycle control, as derived from the KEGG database ( Supplementary Data 2 ). Many polymorphisms and several copy number alterations were found in these genes, sometimes in all of the 293-derived lines but mostly in just a few of them. Almost all polymorphisms were heterozygous and those that were homozygous were very unlikely to be drivers of the transformed phenotype of the cells because of their common occurrence in the human population. We conclude that the adenoviral insertion at high copy number, possibly in conjunction with low fumarate hydratase copy number, is possibly the only main driving factor for the transformed phenotype of the 293 cell lineage in general. We identified a set of 136 genes that were consistently differentially expressed ( P <0.01 and at least twofold change) upon pairwise comparison of each derivative 293 line with the parental 293 line ( Fig. 1b , Supplementary Figs 6 and 7 and Supplementary Data 5 ). The bulk of these genes are involved in cell adhesion and motility, or the regulation thereof. This is commensurate with the phenotype of the parental 293 line, which is generally more difficult to dissociate from culture dishes than the other lines. In addition, we observed a pattern of up- and downregulated genes that is consistent with cell cycle activation and proliferation ( Supplementary Figs 6a,b and 7b and Supplementary Data 5 ), which is in agreement with the observation that the 293 derivative lines used in our study grow much faster than the parental 293 line. This finding indicates that the cell lines derived from the original 293 lines have further been selected through extensive in vitro cultivation for rapid growth under these conditions, and evidence for this is found in the genome of these lines. Examples include the upregulation of MYC and MIR17HG (miR-17-92 or ONCOMIR1 ), the downregulation of CDKN1A , IFI16, BMP2, RPRM and the differential expression of a set of genes resulting in a general TGFβ pathway downregulation [27] in derivative 293 lines compared with the parental 293 line. These genes also influence each other in their expression [28] , [29] , [30] . Sublineage-specific transcriptional alterations, in particular those related to the partial epithelial–mesenchymal transition signature of the 293S-lineage lines, are elaborated on in Supplementary Fig. 8 . Although MYC expression was higher in each of the 293 lines compared with the parental 293 line, we only observed a focal amplification of a 1,500-kb region encompassing the MYC locus in the 293S line ( Fig. 3a ), resulting in a copy number of five compared with a copy number of two or three in the other lines. Consistently, the increase in MYC RNA levels, comparing with the parental 293 line, is stronger in the S line (11-fold) than the SG line (eightfold) and the T and FTM lines (around fourfold), a pattern confirmed using quantitative RT-PCR (RT-qPCR; Fig. 3b ). In addition, this genomic region concurs with flanking interchromosomal rearrangement breakpoints involving chr19 and chrX, indicating that the MYC amplification is because of distal duplication, accompanying translocations. Figure 3: Notable amplifications and deletions in 293 cell lines. ( a ) On the q-arm of chromosome 8, the 293S line shows an amplification of a 1.6-Mb region containing the MYC locus. The 293SG and 293SGGD lines seem to have partially lost this rearrangement. ( b ) Expression validation by quantitative real-time PCR for MYC and three microRNAs from the polycistronic MIR17HG locus (mir17, mir20a and mir92a, respectively). Expression levels of these microRNAs are markedly higher in 293T than in any of the other 293 lines (fold change between 2.5 and 8.8). Values are represented as normalized relative quantities (NRQ)±s.e.m. ( n =3). Significantly different NRQs in comparison with the 293 line are indicated as * P value<0.05, ** P value<0.01, *** P value<0.001 and were analysed using a one-way analysis of variance with a Tukey HSD post hoc test. ( c ) Similarly, the MIR17HG gene is located in an extended amplified region on chr13 in the 293T cell line, where copy numbers reach up to 8. ( d ) Part of the LRP1B gene—comprising exons 3–7 (300 kb) or 4–7 (400 kb)—has been deleted in the 293FTM and 293T line. Copy numbers downstream of this region are also reduced in 293FTM. See also Supplementary Fig. 5 for another notable deletion (including fumarate hydratase, found in all investigated 293 cell lines). In panels a , c and d , the Y-axis represents the genomic copy number. Full size image Likewise, MIR17HG is located in a 7-Mb region that is focally amplified in 293T ( Fig. 3c ), resulting in approximately seven copies. Using RT-qPCR, we validated that microRNAs encoded by the MIR17HG cluster had markedly higher expression levels in 293T than in the other 293 lines ( Fig. 3b ). The 293T line overexpresses the SV40 T protein [8] , [9] , which forms a complex with and inhibits p53, thereby compromising genome integrity [10] . In keeping with this, taking the 293 genome as a baseline, we find more novel structural variants (SVs) in the 293T line than in the other derived lines: 172 versus 89, 95, 92 and 106 for 293FTM, 293S, 293SG and 293SGGD, respectively. In the 293T and 293FTM lines, we observed a homozygous deletion affecting exons 4–7 of the tumour suppressor LRP1B gene ( Fig. 3d ), as well as heterozygous deletions in the flanking regions. Functional loss of LRP1B is implicated in a variety of human cancers [31] , [32] , [33] , [34] through an as yet poorly understood mechanism [35] . The genomic steady state of 293 cell lines To investigate whether 293 cell lines are in genomic ‘steady state’ when handled using standard procedures for cell cultivation and cell banking, we resequenced the genome of the 293T cells twice more. We chose the 293T cells because the presence of SV40 T inhibits p53 and thus this cell line would be predicted to have the fastest genome structural evolution [10] . First, we froze the sequenced 293T cells in liquid nitrogen and recovered and cultivated them under the same conditions as before the first sequencing, resulting in a total of seven extra passages since the first sequencing experiment. This cell preparation was named 293T_14. Second, we obtained 293T cells from our tissue culture facility, where these cells are produced continuously for use in a multitude of experiments in our department. The cells derive from the same original frozen master cell bank (made in 1996) as the other previously sequenced 293T cells, but through a history of many passages and several freezings as working cell banks. This sample of 293T cells (293T_lab) should reflect what happens to the 293T genome in normal laboratory practice over lengthy periods of time. Genomic DNA was sequenced with CG technology. Using principal component analysis, we analysed the SNP pattern of these 293T cell preparations together with the ones of the previously sequenced 293 cell line genomes. As can be seen in Fig. 4a , the three 293T cell line samples cluster very tightly together in the principal component loading plot, showing that these cell lines are indeed much more closely related to one another than they are to the other 293 cell lines. Furthermore, we compared the 2-kbp-resolution copy number derived from the three 293T samples with each other and with the 293 parental cell line ( Fig. 4b and Supplementary Fig. 9 ). As can be concluded from Fig. 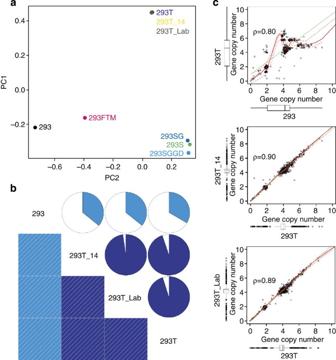Figure 4: Effect of freezing and passaging on 293T genome stability on SNP content, whole-genome CNV and gene copy number. (a) PCA (principle component analysis)-correlated SNP clustering reveals a strong correlation between the different 293T sequencing samples. Notably, this analysis also substantiates the common origin of the S lineage cell lines. (b) Comparison of the genome-wide 2-kb CNV content of the 293T samples among each other and with the 293 line again confirms the high consistency between 293T samples. The darker the shade of blue in the chart, the higher the correlation. (c) Comparison of gene copy number between the various 293T samples and 293. While the copy number of genes in the 293 line considerably deviates from the 293T gene copy numbers, the pattern of gene copy number of the newly sequenced 293T samples is very similar to the sequenced line of lower passage number. 4b , the correlation coefficient between the three 293T genome’s 2-kbp copy number data is greater than 0.87 ( Supplementary Table 4 ), whereas this is again much different when comparing any of the 293T genomes with the one of, for example, 293 cells. We also correlated the copy number of all genes in these different genomes ( Fig. 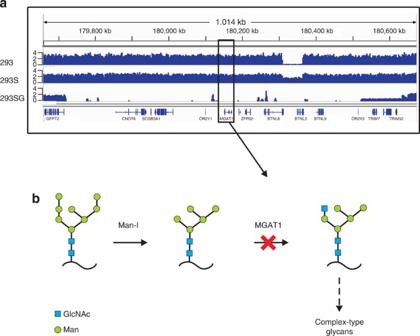Figure 5: Deletion of MGAT1 in 293SG and 293SGGD. (a) Selection for 293S cells without the GnTI activity of MGAT1 using EMS mutagenesis and the ricin toxin induced a 800-kb deletion at the end of chr5. This illustrates that the driving force for mutations in these cell lines are chromosomal rearrangements rather than point mutations. (b) Simplified scheme of early N-glycan processing of glycoproteins in the Golgi apparatus. Loss of MGAT1, responsible for GnTI activity, ensures that N-glycans in the Golgi are committed to the oligomannose type. In panel a, the Y-axis represents the genomic copy number. 4c and Supplementary Table 5 ), which shows again the close similarity between the three 293T genomes. Figure 4: Effect of freezing and passaging on 293T genome stability on SNP content, whole-genome CNV and gene copy number. ( a ) PCA (principle component analysis)-correlated SNP clustering reveals a strong correlation between the different 293T sequencing samples. Notably, this analysis also substantiates the common origin of the S lineage cell lines. ( b ) Comparison of the genome-wide 2-kb CNV content of the 293T samples among each other and with the 293 line again confirms the high consistency between 293T samples. The darker the shade of blue in the chart, the higher the correlation. ( c ) Comparison of gene copy number between the various 293T samples and 293. While the copy number of genes in the 293 line considerably deviates from the 293T gene copy numbers, the pattern of gene copy number of the newly sequenced 293T samples is very similar to the sequenced line of lower passage number. Full size image Furthermore, we used SNP-array analysis for all of the other sequenced cell lines, again upon freezing and multiple passaging. While this analysis provides lower resolution than full-genome resequencing, we again concluded that the genome of these cells is in steady state throughout these common manipulations, except for the 293S line, which showed dramatic copy number alterations upon unfreezing ( Supplementary Data 6 ). In conclusion, these data strongly indicate that the genomic resource for the different 293 cell lines that we provide here will continue to be valid and useful after multiple passaging of the sequenced cell lines, after these are distributed to and cultivated in different laboratories, as long as the cells are handled according to standard cell cultivation procedures. An exception appears to be the 293S line. 293 cell genomic instability under selective conditions One of the engineering steps to derive the 293SG cell line from 293S was an EMS mutagenesis, which is introducing point mutations (in particular through guanine alkylation), followed by selection with the cytotoxic lectin ricin [12] . From the very few resistant clones obtained, one had undetectable N-acetylglucosaminyltransferase I (GnTI) activity. Before the genome sequencing project, we expected to find inactivating GnTI point mutations because of the nature of the mutagenesis method that we used, but instead, a region of ~800 kb at chromosome 5q35.3 has been completely deleted ( Fig. 5a ). This region contains the MGAT1 gene, which encodes the GnTI protein ( Fig. 5b ), and nine other genes unrelated to glycosylation processes. The 800-kb-deleted region is embedded in a much larger region that has undergone massive rearrangements in this clone. Figure 5: Deletion of MGAT1 in 293SG and 293SGGD. ( a ) Selection for 293S cells without the GnTI activity of MGAT1 using EMS mutagenesis and the ricin toxin induced a 800-kb deletion at the end of chr5. This illustrates that the driving force for mutations in these cell lines are chromosomal rearrangements rather than point mutations. ( b ) Simplified scheme of early N-glycan processing of glycoproteins in the Golgi apparatus. Loss of MGAT1, responsible for GnTI activity, ensures that N-glycans in the Golgi are committed to the oligomannose type. In panel a, the Y-axis represents the genomic copy number. Full size image Interestingly, the MGAT1-containing region is the only deleted one in the whole genome and would draw immediate attention for, for example, short hairpin RNA (shRNA)-based candidate gene validation if this were a discovery experiment in which one was looking for the genes underlying resistance to ricin toxin. A tool to detect plasmid insertion sites 293 cell lines are known to contain an adenoviral sequence integration on chromosome 19 (ref. 4 ), and the derived lines (except for 293S) have undergone one or more stable transformations with plasmids. However, we know very little about where and how plasmids insert in the genome. Moreover, one concern with the use of cell lines that have been manipulated for decades in a variety of laboratories is inadvertent contamination with other plasmids or viral vectors. The availability of deep-coverage sequencing data provides an opportunity to investigate these matters. For this analysis, we assembled a database consisting of the vector sequences in the UniVec database build 7.0, expanded with all of the published DNA/RNA virus sequences from RefSeq and completed with the sequences of the plasmids that were used in the transformations to derive the different 293 cell lines sequenced here (details in Supplementary Notes 3 and 4 ). After mapping the sequencing reads of the 293 cell lines to this ‘foreign DNA’ database, we concluded that all known integrated plasmids and the adenoviral sequence characteristic of the 293 lineage were indeed present ( Supplementary Data 7 ). Importantly, at the level of sensitivity afforded here, no other plasmids or viral sequences were detected. The known adenoviral DNA insertion site in the 293 genome [4] served as an appropriate positive control for the optimization of our plasmid insertion discovery workflow. We used the adenovirus C serotype 5 genome (Genbank NC_001405) as a target sequence, as sheared DNA of an isolate of this virus was used originally to derive the 293 line. With appropriate read filtering parameters (details in Supplementary Information ), a high-coverage viral-human genome sequence breakpoint was detected in the PSG4 locus ( Fig. 2a , Supplementary Data 7 and 8 ), in agreement with the published insertion site [4] . Breakpoints were verified by touchdown PCR and Sanger sequencing. We then went on to detect plasmid–chromosome breakpoints for all other plasmids used to generate the different 293 cell lines under study ( Supplementary Data 7 ). We successfully validated a.o. breakpoints for all plasmids in the 293FTM cell line, which are shown as examples here ( Fig. 2b , Supplementary Data 8 ). Publicly accessible resources for the cell biology community To enable resource users to ascertain sequencing depth and quality underlying each variant call, we wanted to visualize the sequencing reads underlying these calls. However, there was a lack of publicly accessible visualization tools for these huge data sets. Therefore, we first designed an easily queried website front (the 293 Variant Viewer, http://www.hek293genome.org/index.php ) for the entire sequence variant database (including 'no call' positions), allowing to quickly visualize whether a sequence of interest has either the reference sequence, unequivocally deviates from it (that is, called variant alleles) or had issues either in the quality of the sequencing data set or in the interpretation of this data set (‘no calls’; Fig. 6a ). A description of the underlying database and the web-based visualization tool can be found in Supplementary Information . Furthermore, from any inspected genomic region in this website, we provided a link to the sequencing read data in the publicly accessible integrative genomics viewer (IGV) [36] ( Fig. 6b ) (see also Supplementary Note 5 for an instruction manual on how to access the data). Apart from allowing to visualize the basis for both ‘calls’ and ‘no calls’, importantly, this integration with IGV provides for seamless visualization of the data together with the wide variety of human genome annotation tracks currently available ( Supplementary Fig. 10 ). This enables rich data mining of 293 genome regions that are of interest to any biological study. 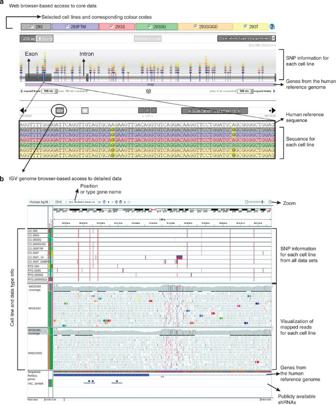Figure 6: Visualization of SNPs and indels in the 293 Variant Viewer. (a) Snapshot of the 293 Variant Viewer for thePIGZgene. The upper region gives an overview of the gene with its variations in each genome, colour-coded by variation type and cell line. Triangles indicate the presence of the variant in a particular genome. The lower part of the browser allows detailed inspection of the sequence and comparison with the human reference genome. A link to the same region in IGV is provided as well. (b) Overview of SNP calling and realignment data tracks in the IGV genome browser for the same gene as ina. The two SNP calling algorithm tracks (CG and RTG) are shown with homozygous SNPs (red bar) and heterozygous SNPs (red/blue). In the CG tracks, no-calls are also shown in light red. In regions where the realignment coverage is zero, the sequence is the same as the human reference sequence. The TRC shRNA track allows the detection of SNPs in target regions of the shRNAs from the TRC2 collection (Broad Institute and Sigma). Mousing-over the different tracks provides users with extra information about specific features, such as mapping quality, base type count and phred scores. Figure 6: Visualization of SNPs and indels in the 293 Variant Viewer. ( a ) Snapshot of the 293 Variant Viewer for the PIGZ gene. The upper region gives an overview of the gene with its variations in each genome, colour-coded by variation type and cell line. Triangles indicate the presence of the variant in a particular genome. The lower part of the browser allows detailed inspection of the sequence and comparison with the human reference genome. A link to the same region in IGV is provided as well. ( b ) Overview of SNP calling and realignment data tracks in the IGV genome browser for the same gene as in a . The two SNP calling algorithm tracks (CG and RTG) are shown with homozygous SNPs (red bar) and heterozygous SNPs (red/blue). In the CG tracks, no-calls are also shown in light red. In regions where the realignment coverage is zero, the sequence is the same as the human reference sequence. The TRC shRNA track allows the detection of SNPs in target regions of the shRNAs from the TRC2 collection (Broad Institute and Sigma). Mousing-over the different tracks provides users with extra information about specific features, such as mapping quality, base type count and phred scores. Full size image As an example, knowledge of the exact target sequence for silencing RNA or genome-editing nucleases would enhance the reliability of such experiments. The 293 genome-sequencing data now afford this resource. We analysed which of the >300,000 Broad Institute mouse/human genome-wide shRNAs mapped uniquely to the human RefSeq gene collection, visualized these in an IGV annotation track ( Fig. 6b ) and investigated which of these targets are mutated in our 293 cell lines. Depending on the cell line, this was the case for 9,608–11,534 (~6% of the ones that aligned) of these shRNAs, which may render these nonfunctional in gene silencing. The 293 line was also one of the many cell lines selected for analysis by the ENCODE project [37] . Several data sets that are highly complementary to ours and deal, for example, with epigenomics are becoming available in this way. We will be updating our web interfaces for the 293 genome with these and other generated data sets on an ongoing basis. Cell lines are instrumental for our growing understanding of mammalian biology and for biopharmaceutical production. 293 cells are second only to HeLa cells in the frequency of their use in cell biology (a search in PubMed for this cell line and its most popular derivatives yields ~20,000 hits). They are second only to CHO cells for their use in biopharmaceutical production (and take the prime spot for use in small-scale protein production and in viral vector propagation). However, 293 cells were at some point derived from an individual human embryo with a genome different from the reference. Moreover, the establishment of the cell line and its continuous growth in vitro impose selective conditions on the cells, which are often adapted to through mutation. Thus, the human reference genome sequence provides only a partial understanding of the genome of human cell lines. As genome-wide short interfering RNA resources are now available for human cells [38] , [39] , and as sequence-specific genome-engineering tools are rapidly becoming standard tools for mammalian cell genetic engineering [40] , [41] , [42] , a sequence and average copy number level knowledge of the entire genomes of the cell lines under study is of great advantage. Furthermore, the cell-line-specific genome sequences reported here will also be beneficial in the interpretation of RNA-seq and proteomics experiments that make use of these cells. 293 cells have been cultivated for decades in different laboratories, which most likely has led to different progressive genome structure alterations. This may underlie the sometimes different conclusions drawn from experimentation with 293 cell lines (and many other cell lines). All cell lines sequenced here are available to the research community. Up to the level of sensitivity afforded by our sequencing approach (single copy plasmid insertions were easily detected), these cell lines have no inadvertent virus insertions, which should help to put at rest some of the concerns towards the use of the 293 cells for biopharmaceutical production. The analytical tools we provide here for integrated plasmids and viral sequences will be very valuable in fully characterizing cell lines used for the production of biopharmaceuticals, both towards the copy number and stability of the inserted plasmids and the validation that such cell lines are free of inadvertent viral sequence contamination. We have shown that comparative sequencing of several 293 lines of the same descent reveal genomic copy number alterations that explain diverse phenotypes of the lineage and its subclones. Extensive further experimentation is now required to validate the role of these CNVs in cellular transformation, suspension growth adaptation and metabolism. We hope that such studies will contribute to the design of new generations of 293 cells that are even better adapted to experimental and pharmaceutical production requirements, and the knowledge gained may be instructive in how to directly engineer other human cell lines. Furthermore, it is clear from our data that the standard practice of generating a stable clone through transfection and selection will result in the isolation of one geno/karyotype present in the parental cell line. Thus, any phenotype of the resulting stable transfectant may be because of the integrated transgene, or may be because of a genomic difference between the new line and its parental line. Consequently, such experiments should be interpreted with great caution and these data argue for the use of efficient transient transfection or propagation of a polyclonal pool of stable transfectants (in which case a more representative population of the parental cells is analysed) in, for example, quantitative signal transduction studies that use 293 cells (as is used in many drug screening and ‘omics’ experiments). However, the other side of the medal is that there is promise in a potential forward genetics approach offered by analysing phenotype-causative focal copy number variations (in particular full deletions) in 293-derived clones selected for adaptation to new growth conditions (such as high-cell density cultivation while producing biopharmaceuticals, virus infection, activation of particular signal transduction pathways and so on). This approach is made possible by the apparent property of 293 cells to have lost control over chromosomal structure to a great extent. Consequently, a culture of 293 cells should be considered as an entire 'population' of individual cells with different chromosomal structure makeup. Copy number variations are easy to identify at high resolution using high-coverage resequencing. Further experimentation will reveal whether phenotype-selected copy number variations can always be distinguished from such variations that occur randomly. In this perspective, genomic diversity of the 293 cell line might prove to be an experimental opportunity and might further enhance its role as a provider of knowledge on human cell biology. Cell cultivation for DNA and RNA preparation All cell lines were cultured from frozen stocks at 37 °C in Dulbecco’s Modified Eagle Medium (DMEM; Invitrogen) supplemented with 10% (v/v) fetal calf serum, 2 mM L -glutamine, 100 U ml −1 penicillin G, 110 mg l −1 sodium pyruvate and 100 μg ml −1 streptomycin. All lines were routinely split twice a week, when ~80% confluency was reached. Depending on the cell line, the dilution was between 1:3 (293A) and 1:20 (293T). To prepare genomic DNA, ~30 million cells were harvested for each line. The genomic DNA was extracted and purified using the Gentra Puregene Cell kit (Qiagen GmbH, Hilden, Germany) with RNAse treatment of the samples, according to the manufacturer’s instructions. DNA concentrations were determined fluorimetrically with the Quant-iT PicoGreen dsDNA Reagent (Molecular Probes, Life Technologies Ltd., Paisley, UK). For RNA preparation, the cell lines were cultured in 75-cm 2 filter cap flasks in a humidified, 8% CO 2 atmosphere incubator in DMEM/Ham’s F12 (DMEM/F12; Invitrogen) supplemented with 10% (v/v) fetal calf serum, 2 mM L -glutamine, 100 U ml −1 penicillin G and 100 μg ml −1 streptomycin. Flask positions in the incubator were randomized daily to correct for potential temperature biases. Total RNA was extracted from three replicates of each cell line using Qiagen’s RNeasy Midi kit according to the manufacturer’s instructions, including an on-column DNase-I digest. Concentrations were determined with a NanoDrop ND-1000 spectrophotometer (Thermo Scientific), and RNA quality was assessed on a 2100 Bioanalyzer using RNA 6000 Pico chips (Agilent Technologies). All samples had an RNA integrity number of 9.5 or better. For the RT–qPCR validation of miRNA expression levels, procedures were identical except that the small RNAs were isolated using the miRCURY RNA isolation kit Cell and Plant (Exiqon), again according to the manufacturer’s instructions. Exon arrays After spiking total RNA from each cell line with bacterial poly-A RNA-positive controls (Affymetrix), every sample was reverse-transcribed, converted to double-stranded cDNA, in vitro -transcribed and amplified using the Ambion WT Expression Kit. The obtained single-stranded cDNA was biotinylated after fragmentation with the Affymetrix WT Terminal Labeling kit as outlined in the manufacturer’s instructions. The resulting samples were mixed with hybridization controls (Affymetrix) and hybridized on GeneChip Human Exon 1.0 ST Arrays (Affymetrix). The arrays were stained and washed in a GeneChip Fluidics Station 450 (Affymetrix) and scanned for raw probe signal intensities with the GeneChip Scanner 3000 (Affymetrix). For the processing of the data, see extended experimental procedures. Exon-array data analysis We used a combination of the R Statistical Software Package ( www.r-project.org ) and Affymetrix Power Tools (APT; Affymetrix) for the quality control and differential expression analysis of the exon-array data, partly as described earlier [43] . The full R code and APT commands are available as in Supplementary Data 9 and 10 ). Briefly, exon- and gene-level intensity estimates were generated by background correction, normalization and probe summarization using the robust multi-array average algorithm with APT. At the gene level, after quality control of the raw data in R, genes of which the expression was undetected in all six lines were removed from further analysis, as were the genes of which expression was below the estimated noise level in all lines. This noise level threshold was set at the signal intensity level that eliminated ‘detection’ of expression of more than 95% of the genes on the Y-chromosome, which is absent from the HEK293 lineage (which was derived from a female embryo) and thus serves as an appropriate internal negative control. Differential gene expression analysis was performed for the relevant cell line pairs using a linear model fit implemented in the R Bioconductor package Limma [44] , considering only core probe sets. The Benjamini–Hochberg (BH) method was applied to correct for multiple testing. Lists of significantly up- and downregulated genes (BH-adjusted P values<0.01) with a minimal twofold change in expression were subjected to functional enrichment analysis using DAVID [45] and IPA (Ingenuity Systems, www.ingenuity.com ), transcription factor regulation prediction using DiRE [46] and manual inspection. Those lists are available as Supplementary Materials . For integration in the IGV genome browser [36] , we chose to display all genes found to be differentially expressed (BH-adjusted P value<0.01) in the pairwise comparison of interest, irrespective of their log2-fold change, which is displayed as a function of the bar height. The ‘web link to gene expression data’ track links every gene of which expression was detected to a table with the statistical details. The mean exon expression values in the IGV ‘mean probe set expression’ tracks represent the log2 signal values of the filtered extended exon probe sets, that is, after removal of undetected, cross-hybridizing and noisy probes. CG sequencing and analysis Anticipating the pseudotriploidy of the HEK293 genome, genomic DNA from each cell line was submitted to CG’s sequencing service [16] (detailed in Supplementary Information ) with the request to maximize the sequencing machine’s output to achieve the highest coverage possible, yielding 158~287 Gb of mapped reads of which 122~190 Gb of reads mapped with an expected paired distance ( Supplementary Tables 1 and 2 ). The raw data were analysed with version 1.11 of the company’s analysis software and processed with CGAtools v1.5 ( http://cgatools.sourceforge.net/ ). This pipeline entails read mapping followed by local reassembly of reads that map to a region in which deviation from the reference sequence is suspected from the mapping results. This is then used as the input for SNP and small indel calling. A second analysis focuses on copy number variation (see Supplementary Note 1 ) and uses the genome-normalized average sequence coverage as input, together with the genome-normalized sequence coverage of 46 normal diploid human genome-resequencing data sets (baseline genome) for the area under analysis. These latter data are used to correct the coverage for sequence-specific biases in the sequencing workflow. The output of this analysis is 2-kbp-resolution copy number expressed as a factor relative to a copy number of 2. As described in the main text, we derived true copy number from these data through calibration with genome-weighted average ploidy as derived from Illumina SNP-array data ( Supplementary Table 6 ). A third analysis uses the paired-end reads of which the mate pairs do not map to a continuous stretch of the human reference genome sequence, and which thus provide evidence for chromosomal rearrangements. These reads are de novo assembled into ‘junction sequence contigs’ that contain the information about the breakpoints involved in such chromosomal rearrangements. The CG raw data and initial analysis results were processed by CGAtools v1.5 ( http://cgatools.sourceforge.net/ ) with scripts from the CG user community tool repository and our in-house scripts (see Supplementary Note 2 ). To enable independent analysis of the data, we mapped the sequencing reads to the human reference genome, build hg18, using RTG Investigator from Real Time Genomics ( http://www.realtimegenomics.com/ ) with default setting (maximum mate-pair insert size: 1,000, minimum insert size 0 and report the maximum best five matches). Upon mapping, SNP and small indel calling were also performed using the RTG software Investigator. Only SNP/indels passing the quality filter (called in more than half of the reads and covered by less than 200 × coverage to avoid variant calling in highly repetitive regions) were kept for further analysis. The lists of SNPs and indels called either by CG or RTG were merged by vcftools [47] . To remove platform-specific artifacts from the CG sequencing, the extended variant list was filtered using ANNOVAR [48] , to remove variants located in a region where less than 30% of the CG69 data sets had sequencing information. We then functionally annotated this filtered extended variant list by ANNOVAR. We used GenomeComb ( http://genomecomb.sourceforge.net/ ) to reformat the SNV calling results from CG for the six cell lines [49] . In order to increase the number of concordants between cell lines and reduce the false-positive SNV calling rate, we used the obligatory filtering strategy: remove uncertain calls and filtered based on the variant score reported from CG in each cell line. Variant scores lower than the reported average variant score were removed. The SVs detected from CG analysis were first filtered with cgatools against the publicly available Yoruban (NA19238) CG genome data set, to remove frequently occurring SVs. SVs in the 293-derived cell lines were further filtered against the 293 line and we only retained those with low frequency (<10%) in the CG69 population for further manual inspection. SNP-array procedures Genomic DNA (same sample as used for genome sequencing) of each cell line was analysed using the Illumina HumanCytoSNP-12 v2.1 SNP-array, entirely according to the manufacturer’s instructions. For analysis, we used the ASCAT algorithm, which accurately determines allele-specific copy numbers in tumours and aneuploid cell lines by estimating and adjusting for overall ploidy and effective tumour fraction in the sample [50] . ASCAT uses the raw BAF and logR data of the Illumina HumanCytoSNP-12 v2.1. Accession codes: Complete Genomics sequencing data have been deposited in the European Nucleotide Archive (ENA) under the accession code PRJEB3209 . The Affymetrix exon-array data have been deposited in the ArrayExpress Archive under the accession code E-MEXP-3516 . How to cite this article: Lin, Y.-C. et al. Genome dynamics of the human embryonic kidney 293 lineage in response to cell biology manipulations. Nat. Commun. 5:4767 doi: 10.1038/ncomms5767 (2014).